Reactant-induced photoactivation of in situ generated organogold intermediates leading to alkynylated indoles via Csp2-Cspcross-coupling Photosensitization of organogold intermediates is an emerging field in catalysis. In this context, an access to 2,3-disubstituted indoles from o -alkynyl aniline and iodoalkyne derivatives via a gold-catalyzed sequence under visible-light irradiation and in the absence of an exogenous photocatalyst was uncovered. A wide scope of the process is observed. Of note, 2-iodo-ynamides can be used as electrophiles in this cross-coupling reaction. The resulting N -alkynyl indoles lend themselves to post-functionalization affording valuable scaffolds, notably benzo[a]carbazoles. Mechanistic studies converge on the fact that a potassium sulfonyl amide generates emissive aggregates in the reaction medium. Static quenching of these aggregates by a vinylgold(I) intermediate yields to an excited state of the latter, which can react with an electrophile via oxidative addition and reductive elimination to forge the key C-C bond. This reactant-induced photoactivation of an organogold intermediate opens rich perspectives in the field of cross-coupling reactions. In the quest of synthetic efficiency featuring notably step economy, dual catalysis through the merger of transition metal-catalysis and photocatalysis has constituted undoubtedly a major advance [1] , [2] , [3] . As early as in 2007, Osawa observed an acceleration of a copper-free palladium-catalyzed Sonogashira coupling in the presence of Ru(bpy) 3 (PF 6 ) 2 [4] . It was claimed that the latter facilitates the oxidative addition step but no mechanistic evidence was provided. In 2011, the Sanford group highlighted that the photoreduction of an aryldiazononium salt via single electron transfer (SET) could be coupled to a Pd(II)/Pd(IV) manifold involving a directed C–H activation to provide bis-aryl products. The design of these transformations relied on the intertwining of a photoredox cycle with the palladium cycle, which ensures the adequate electronic shuttle [5] . This seminal report launched the field of metallaphotocatalysis [1] which found valuable applications, notably in gold(I) catalysis a fertile field of investigations over the last two decades [6] , [7] . Indeed, in order to access to higher molecular complexity [8] , [9] , the frequently encountered protodeauration step has to be circumvented and the post-functionalization of organogold intermediates [10] via C–C bond formation appears highly desirable. Nevertheless, in contrast to the commonly used metals in catalysis and due to the high redox potential of the Au(I)/Au(III) couple [11] , the oxidative addition at gold(I) is difficult. Initial reports have focused on the use of a stoichiometric oxidant [12] , [13] and there has been a need to devise new pathways to promote it [14] , [15] , [16] , [17] . While ligand design for gold(I) has emerged as a possibility [18] , versatile catalytic cross-coupling reactions, notably thanks to the use of hemilabile (P,N) ligands, have been recently worked out [19] . In addition, Au(I)/Au(III) cycles have also been sustained via photoredox catalysis using aryl-diazonium or iodonium partners as SET partners [13] , [20] , [21] , [22] , [23] . Synthetically relevant sequences have resulted but the question to know how those actually work is still pending, notably because some of these reactions proceed in photocatalyst-free conditions [24] , [25] , [26] , or even under irradiation-free conditions in the simple presence of a mineral base [27] . Recently, we have reported a new reactivity paradigm by providing the first example of an energy transfer promoted oxidative addition at gold(I) [28] , [29] . Upon visible-light irradiation, an iridium photocatalyst triggers via triplet sensitization the oxidative addition of an alkynyliodide onto a vinylgold(I) intermediate to deliver Cs p 2 -C sp coupling products after reductive elimination. Mechanistic and modeling studies suggest that no redox pathway is involved but that an energy transfer [30] , [31] , [32] takes place to generate a triplet state of the vinylgold intermediate. The latter can engage in an oxidative addition with an alkynyl or a vinyl iodide. This mode of activation in gold homogenous catalysis was applied in several dual catalytic processes. For instance, alkynylbenzofuran derivatives like 3- O could be obtained from o -alkynylphenol 1- O and iodoalkyne 2a in the presence of a catalytic mixture of a gold(I) ( [AuCF 3 ] : ([( p -CF 3 Ph) 3 PAuCl]) and an iridium(III) complex ([Ir[dF(CF 3 )ppy] 2 (dtbbpy)PF 6 ]) under blue LEDs irradiation (Fig. 1a ). Fig. 1: Gold(I) catalysis under visible-light. a Previous work [28] : alkynylative cyclization of o -alkynylphenols via phosensitized oxidative addition. b Contrasting reactivity between the phenol and the sulfonamide precursors 1- O and 1a . Full size image While we were studying possible synthetic extensions of this chemistry, we made some puzzling observations when comparing the reactivity of o -alkynylphenol precursor 1- O vs. o -alkynyl N -tosylamide 1a . In iridium-free conditions, but in the presence of 5 mol% [AuCF 3 ] and K 2 CO 3 under blue LEDs irradiation, only a very little amount of 3- O (5%) was observed (Fig. 1b ). In sharp contrast, these iridium-free reaction conditions proved to be perfectly suited for the formation of indole 3aa (64% yield) from NTs amide 1a . Structures of 1a and 3aa were confirmed by X-ray diffraction (XRD) analysis. In this work, the generality of this reaction is examined since indoles are key motifs in many relevant natural products and are also privileged scaffolds in medicinal chemistry, agrochemical industry, personal cares as well as dyes [33] , [34] , [35] . It is also the occasion to investigate the mechanism and notably how the heteroatomic nucleophilic component ( N - vs. O -nucleophile) alters the photochemical activation process in these exogenous photocatalyst-free transformations. 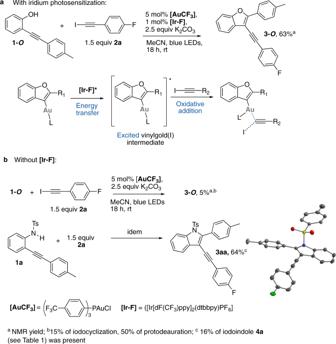Fig. 1: Gold(I) catalysis under visible-light. aPrevious work28: alkynylative cyclization ofo-alkynylphenols via phosensitized oxidative addition.bContrasting reactivity between the phenol and the sulfonamide precursors1-Oand1a. Optimization of the conditions We screened some variations on the reaction parameters in order to check if we were working in the most favorable set of conditions (Table 1 ). We first checked that the use of PPh 3 AuCl (entry 1) instead of [AuCF 3 ] was detrimental for the reaction since only 50% of conversion was observed and only 8 % of 3aa was detected on the crude 1 H NMR spectrum, accompanied by 10% of iodoindole 4a as iodocyclization by-product. The addition of 1 mol% [Ir-F] was productive in 3aa but not as much as in photosensitizer free conditions (38% vs. 64%, entries 2 and 4) and the selectivity 3aa vs. 4a was lower. The addition of 10 mol% benzophenone as photosensitizer proved to have no effect in terms of yield and selectivity for 3aa (entry 3). In order to reduce the quantity of 4a , we diminished the source of iodine (iodoalkyne 2a ) in the reaction conditions. Engaging a 1:1.1 ratio of 1a and 2a (entry 5) proved to be as yielding as previous conditions (1:1.5 ratio, entry 4) but more selective toward 3aa . Variation of the counter ion gave contrasted results and confirmed the supremacy of the potassium cation over sodium (entry 6), cesium (entry 7) and calcium (entry 8), all three resulting in poor or no conversion. Addition of 18-C-6 caused a consequent yield decrease (only 14% of 3aa , entry 9). While we showed that the reaction could be run by using a preformed potassic salt 1a-K resulting from the deprotonation with KH of 1a (50% of 3aa , Fig. 2a ), addition of 18-C-6 was also deleterious in that case (35% of 3aa accompanied by 10% of protodeauration product 5a ). 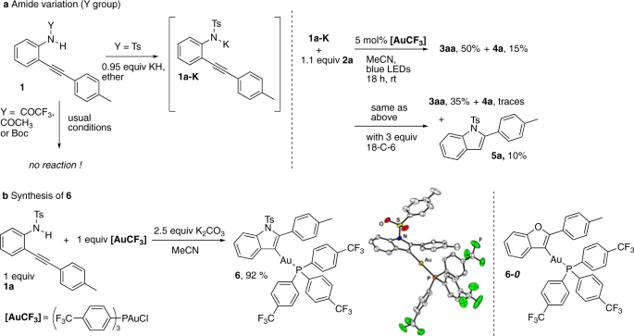Fig. 2: Preparation of putative intermediates and scope. aPreforming the potassic salt1a-Kis possible to obtain the cross-coupling reaction. Of note, whatever the reaction conditions, no product was observed with an amide or a carbamate precursor.bSynthesis of6and its XRD structure. All attempts with an amide (acetamide, trifluoroacetamide) or a carbamate (Boc) precursor failed to give any product. Of note also, no productive reaction leading to 3aa was obtained from the corresponding bromoalkyne 2a-Br and the chloroalkyne 2a-Cl . Overall, this series of findings confirmed us in using a sulfonamide nucleophile and a potassium base in MeCN (see also Supplementary Table 1 ) for further developments. Table 1 Optimization of the formation of indole 3aa. Full size table Fig. 2: Preparation of putative intermediates and scope. a Preforming the potassic salt 1a-K is possible to obtain the cross-coupling reaction. Of note, whatever the reaction conditions, no product was observed with an amide or a carbamate precursor. b Synthesis of 6 and its XRD structure. Full size image Mechanistic studies In order to extend the scope of possible substrates, we wished to get some insight into the mechanism of this transformation. 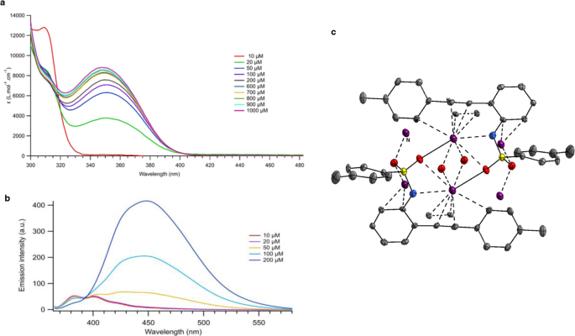Fig. 3: Characterization of 1a-K. Dependence from the concentration of1a-Kin MeCN at 298 K.aOn the molar absorption coefficient.bOn the luminescence spectrum.cXRD structure of1a-K. Red atom: O, yellow atom: S, blue atom: N, purple atom: K. The fact that a photo-triggered event occurs without any photocatalyst logically led us to consider the optical properties of the different partners present in the reaction medium. UV–vis absorption spectra were first recorded (Supplementary Figs. 1 and 2 ) and evidenced that the starting materials 1a and 2a as well as the cross-coupling product 3aa at 50 μM were unable to absorb the light of the blue LED used ( λ max = 450 nm). Species presumably formed in situ were also studied such as vinylgold(I) intermediate 6 . The latter was smoothly obtained in 92% yield by reacting an equimolar mixture of 1a and [AuCF 3 ] in the presence of K 2 CO 3 in MeCN (Fig. 2b ). Crystals were collected and allowed a XRD analysis. Tosylamide anion 1a-K , supposedly originating from the deprotonation of 1a (pKa ≈ 10) in the basic medium was also examined. Complex 6 did not exhibit absorption above 400 nm at 50 μM and comparison between 6 and 6- O showed both vinylgold(I) intermediates exhibit a similar absorption profile (Supplementary Fig. 3 ). In contrast, vinylgold 6 proved much more emissive than 6- O , exhibiting a wide emission band at 400 nm (Supplementary Fig. 4 ). Thorough analysis of the photophysical properties of 1a-K provided important information. First, we observed a dependence of the absorption properties on the concentration of 1a-K . Indeed, by increasing the latter from 10 µM to 1 mM (Fig. 3a and Supplementary Fig. 5 ), the narrow absorption band at 310 nm collapsed and the appearance of a new wide band centered at 350 nm was observed. Second, upon increasing 1a-K concentration, the emission band at 383 nm dropped at the benefit of a wide emission band centered at 450 nm (Fig. 3b and Supplementary Fig. 8 ). All these findings are in line with the formation of aggregates of 1a-K , which could account for chromatic alteration and excimer formation in a regime of strong coupling between the chromophores [36] . In contrast, no such phenomenon was found with a potassic phenolate salt (Supplementary Fig. 6 ). Fig. 3: Characterization of 1a-K. Dependence from the concentration of 1a-K in MeCN at 298 K. a On the molar absorption coefficient. b On the luminescence spectrum. c XRD structure of 1a-K . Red atom: O, yellow atom: S, blue atom: N, purple atom: K. Full size image XRD analysis of 1a-K strengthened both the idea of the formation of aggregates and the crucial role of the potassium counterion since it revealed that each potassium cation is octacoordinated (Fig. 3c ). Besides the electrostatic interaction with the N atom, each potassium connects to four oxygen atoms of four distinct sulfonamide anions and also to two alkyne moieties through η 2 -slipped complexes featuring 3.0973–3.2589 Å and 3.3117–3.1062 Å distances. Such η 2 -slipped complexes remain rare [37] , [38] , but have been invoked in some reactions [39] . The last interaction consists in a η 1 -coordination between a carbon of the tolyl ring and the potassium cation with a distance of 3.3074 Å [37] . Conversely, one can understand the detrimental effect of 18-C-6 that would prevent the formation of this aggregate. Liquid-state NMR experiments were conducted to monitor the aggregation of 1a-K in solution. First, the 1 H NMR spectra at concentrations ranging from 10 to 0.05 mM were recorded (Supplementary Fig. 44 ). It was observed that upon decreasing the concentration, the four proton signals of the di- ortho substituted aniline ring broaden and shift. At 0.05 mM, these broadened signals are at the same chemical shifts than those in pure 1a . These observations are consistent with monomeric 1a-K at that low concentration. Hydrogen (in 1a ) and potassium (in 1a-K ) atoms being similarly bounded to nitrogen, quadrupolar potassium (spin 3/2) alone generates signal broadening. The improvement of the signal resolution by increasing the concentration suggests that the molecules adopt progressively a different spatial organization. This is confirmed by acquiring NOE-1D experiments with 0.05, 0.5 and 10 mM solutions of 1a-K . Clear dipolar interactions are observed between the ortho -aromatic proton of the tolyl group at 7.4 ppm with the two aromatic protons of the tosyl group at 7.2 and 7.7 ppm for 1a-K at 0.5 and 10 mM, while none exists at 0.05 mM (Supplementary Fig. 45 ). Such intermolecular contacts are in agreement with the XRD structure proposed in Fig. 5 . Finally, the self-diffusion coefficient of 1a-K was determined at various concentrations (10, 5, 1, 0.5, 0.1 and 0.05 mM) in acetonitrile-d 3 solutions at 295 K by the PGSE-NMR technique (Supplementary Fig. 46 ). 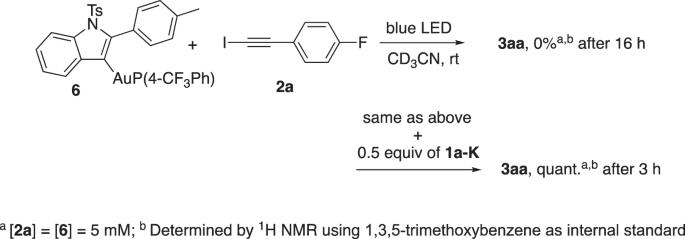Fig. 4: Impact of 1a-K on the direct irradiation of a mixture of 6 and 2a under blue LED irradiation. The presence of1a-Kis necessary to obtain the indole cross-coupling product3aafrom the preformed vinylgold intermediate6. Its value drops from the most diluted to the most concentrated solution, which suggests the formation of aggregates in compliance with the substantial increases of the estimated hydrodynamic radii and molecular weight (Supplementary Table 4 ). The presence of the iodoalkyne 2a does not alter the absorption properties of 1a-K (Supplementary Fig. 10 ). Nevertheless, we observed by 19 F NMR a significant shift of the peak associated to the fluorine atom of 2a upon its titration by a related potassic amide 1g-K at constant concentration of 2a (Supplementary Fig. 11 ). This observation may suggest that 1g-K and 2a yield a complex engaged in a fast exchange with the free species. 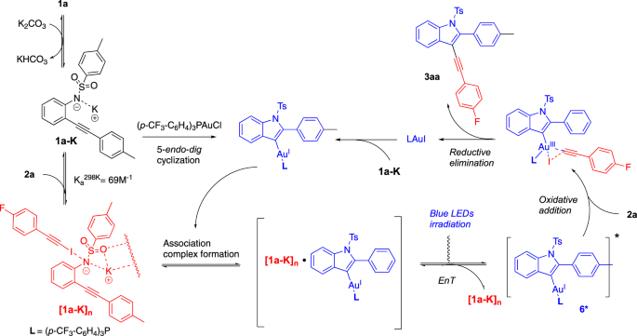Fig. 5: Synoptic mechanism. The blue light-excited1a-Kaggregates in contact with the vinylgold6promote direct Dexter energy transfer. After intersystem conversion, triplet state6*undergoes oxidative addition to iodoalkynes2. Reductive elimination liberates indoles3. 1 H and 13 C NMR analyses corroborated this finding (see Supplementary Figs. 12 and 13 ). We obtained a satisfactory fit of the data by applying a 1:1 association model and retrieved K a 298K = 69 M −1 for the 1g-K : 2a complex association constant at 298 K (Supplementary Fig. 14 ). This value is consistent with the results of Goroff and Diederich [40] , who reported halogen bonding between amines and iodoalkynes of type 2 [41] , [42] . In contrast no such interaction was observed between 1a-K and 2a-Br and 2a-Cl (Supplementary Figs. 15 – 24 ), which is consistent with the order of halogen bonding donor ability I > Br > Cl [42] , [43] . DFT calculations also supported the formation of an halogen bond between 1a-K and 2a and 2b (Supplementary Figs. 38 – 40 ). By analogy with the phenol case [28] , we investigated the reaction of vinylgold 6 with iodoalkyne 2a under blue LEDs irradiation. Thus, at 5 mM which is close to the maximum concentration of 6 in the preparative reactions (i.e. 3.3 mM of gold species, based on 0.3 mmol of 1a and 5 mol% of [AuCF 3 ] in 4.5 ml of MeCN, Supplementary Discussions II. 1. d.) almost no cross-coupling took place, since only traces of 3aa were observed after 16 h of reaction (see Fig. 4 and Supplementary Figs. 25 – 27 ). This observation marked a sharp contrast with the one-pot reaction of entry 5 of Table 1 that smoothly delivers 3aa . We surmised from these findings that a component formed in the reaction medium must promote the transformation. In view of the preceding series of experiments, we raised our suspicions on intermediate 1a-K . Indeed, running the same NMR monitoring experiment in the presence of 0.5 equiv of 1a-K vs. 1a and 6 revealed a contrasting evolution of the reaction (Supplementary Figs. 28 and 29 ). As early as after 10 min, 17 % of 3aa was formed, 45% of 3aa after 0.5 h. After 3 h, the NMR yield reached 100% of 3aa , based on the limiting one equivalent of 2a . Two reactions can contribute to this yield. The first one would consist in the reaction of the vinylgold 6 photoexcited by 1a-K with 2a that also liberates ( p -CF 3 Ph) 3 PAuI (see below). The latter can in turn catalyze the reaction of 1a-K with 2a , which also contributes to the formation of 3aa . As an additional hint of a photosensitization pathway: direct irradiation of a mixture of 2a and 6 in more concentrated conditions (20 mM) yields a rapid reaction leading to 3aa , see Supplementary Figs. 25 and 30 . Fig. 4: Impact of 1a-K on the direct irradiation of a mixture of 6 and 2a under blue LED irradiation. The presence of 1a-K is necessary to obtain the indole cross-coupling product 3aa from the preformed vinylgold intermediate 6 . Full size image To gain further insight into the mechanism, we investigated the impact of 6 on the steady-state luminescence of the 1a-K aggregate excited at 380 nm. We observed a marked luminescence drop when the concentration of 6 was increased (Supplementary Fig. 31 ). Stern–Volmer analysis yielded a slope equal to 9.4 × 10 3 mol −1 l at 298 K (Supplementary Fig. 32 ). To properly interpret this value, we showed that the lifetime of 1a-K* was below 20 ns (Supplementary Fig. 33 ), which suggests that the excited aggregated 1a-K* is a singlet state. Hence, by assuming the quenching to be dynamic [28] , one would extract k Q 298K = 4.7.10 11 l mol −1 s −1 as the lower limit of the rate constant of 1a-K* fluorescence quenching [44] . However, this value is significantly higher than the second-order rate constant for a reaction under control of the solvent diffusion evaluated to k MeCN 298K = 1.8 10 10 l mol −1 s −1 (Supplementary Discussions II. 1. e.) [45] , [46] . To further eliminate the possibility of a dynamic quenching, we showed that a drop of the temperature increased the quenching efficiency (Supplementary Fig. 34 ): the slope of I/I 0 ([ 6 ]) continuously increases from 1.8 × 10 3 l mol −1 at 25 °C to 6.3 × 10 4 l mol −1 at 0 °C. This could not be explained by a quenching under control of diffusion since the solvent viscosity increases when the temperature drops. Therefore, we concluded the quenching to be static and associated to the formation of a non-emissive complex between the 1a-K aggregate and 6 . The slope of the Stern–Volmer analysis was interpreted as the thermodynamic association constant at 25 °C [44] and its temperature dependence was analyzed with the Van’t-Hoff equation to retrieve Δ r H ° = −106.2 kJ mol −1 and Δ r S ° = −299.44 J mol −1 K −1 for the enthalpy and entropy of the 1a-K : 6 complex formation respectively (Supplementary Figs. 35 and 36 ). Interestingly, the luminescence quenching of a 1a-K:2a mixture by 6 even showed a higher slope and allowed to determine a fourfold higher association constant of 1a-K : 2a with 6 (Supplementary Fig. 37 ), which is consistent with a cooperative effect of halogen bonding between the amide and the iodoalkynes, this effect being absent in the case of a bromo- or a chloroalkyne. This would transpose in the reaction medium in such a way that the blue light-excited 1a-K aggregates in contact with the vinylgold 6 would promote direct Dexter energy transfer. Further intersystem conversion would yield the triplet state 6* , which undergoes oxidative addition to iodoalkynes 2 (see Fig. 5 and Supplementary Fig. 41 ). After reductive elimination, the liberated LAuI could promote another catalytic cycle. In addition, DFT calculations supported the whole catalytic cycle and notably the photosensitized oxidative addition through bending of the iodoalkyne partner (Supplementary Fig. 41 ). Fig. 5: Synoptic mechanism. The blue light-excited 1a-K aggregates in contact with the vinylgold 6 promote direct Dexter energy transfer. After intersystem conversion, triplet state 6* undergoes oxidative addition to iodoalkynes 2 . Reductive elimination liberates indoles 3 . Full size image This cross-coupling process enters the examples of photochemical transformations under visible-light for which no exogenous photocatalyst is required to observe a photochemical activation. Several synthetic processes have been shown to follow such pathways and a large part of them have involved photoactive reactants or products [47] , electron donor-acceptor complexes [48] , [49] , [50] or the in situ generation of visible-light absorbing intermediates [51] . Herein, the aggregation of one reactant is the trigger for reactivity. This type of activation remains poorly described and the most closely related example is the aggregation-induced photoreaction of 1,2-diisocyanoarenes [52] . Scope of the reaction Having determined the activation process that governs these transformations, we studied the scope of the reaction. We first varied the alkynyl iodide partners 2 (Fig. 6 ). The reaction proved to be workable on a series of arylalkyne substrates bearing a donor group on the aromatic ring (67% of 3ad and 63% of 3ae , both of them bearing a methoxy group) or with an electron-withdrawing group (56% of 3ai with an ester group, 58% of 3aj with a CF 3 group). In contrast, an alkyl chain on the alkyne gave a more modest yield ( 3ak , 38%). Fig. 6: Scope of alkynes. The reaction works well with arylalkyne substrates 2 bearing a donor group or an electron-withdrawing group on the aromatic ring. In contrast, an alkylalkyne gave a more modest yield. Full size image The aniline platform 1 could also be modulated (Fig. 7 ). Variation of the alkynyl substituent R 1 was first examined. When dealing with an aromatic alkyne, no much yield variation was observed since most yields of products 3 were above 60% even with more contrasting electronic demand (64% of da and 68% of db with a 4-methoxy group vs. 60% of 3ib with a 4-CF 3 group). Of note, the presence of a 4-methoxy group on the aromatic ring did not significantly result in protodeauration on the contrary to our previous arylative cyclization of O -alkynyl phenols [28] . While for R 1 = H no conversion was observed, donor alkyl groups on the alkyne proved also competent providing 2-alkyl indoles 3ja (R 1 = Me, R 2 = F), 3 kb (R 1 = n -Pent, R 2 = H) and 3 lb (R 1 = 4-Cl- n -Bu) in respectively 59%, 58% and 49% yields. Introduction of a chlorine or a methyl group in 4-position of the aniline precursor gave average yields (<50%) of products 3mb and 3nb . We also wished to survey the importance of a sulfonyl group attached on the nitrogen atom of the aniline precursor by varying the R 3 group. In general more modest yields of indole products were obtained with mesylate precursors that gave the corresponding products 3Ms-aa in 32% yield or 3Ms-ab in 37% yield. Although the N -detosylation of indoles is known [53] , even more easily disposed sulfonamide groups were tested and 42% of nosyl-indole 3Ns-aa and 45% of 2-(trimethylsilyl)ethanesulfonyl (SES) indole 3SES-aa were obtained. The latter could be easily converted into the free NH indole 3aa-H by treatment with Bu 4 NF as shown in Fig. 7 . Fig. 7: Scope of anilines. The reaction is compatible with a large scope of alkyne R 1 substituents (aryl or alkyl). A methyl group on the alkyne is even possible ( 3ja ). Variation of the sulfonyl group is possible. Easily removed nosyl (Ns) and 2-(trimethylsilyl)ethanesulfonyl (SES) groups are compatible with the reaction. Full size image In order to extend the synthetic scope of this process and also to provide substrates for valuable post-functionalizations, we focused our attention on 2-iodo-ynamide 7 as an electrophilic partner (Fig. 8 ). Interestingly, this substrate has been only described once by Danheiser who used it as a [2 + 2] cycloaddition partner [54] . From a broader perspective, very few examples of metal-catalyzed cross-coupling of such halo-ynamides have been published, all of them from bromo- or chloro-ynamides with copper [55] , [56] , [57] but none with gold. 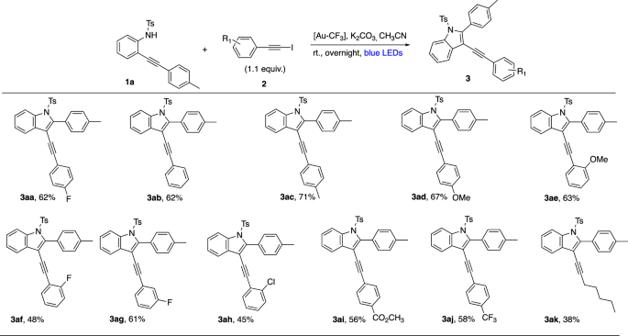Fig. 6: Scope of alkynes. The reaction works well with arylalkyne substrates2bearing a donor group or an electron-withdrawing group on the aromatic ring. In contrast, an alkylalkyne gave a more modest yield. 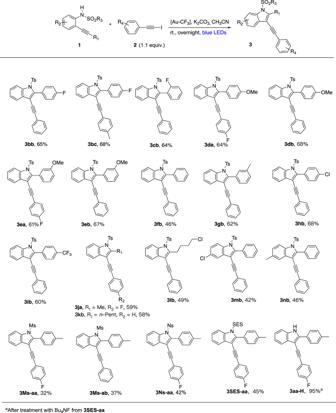Fig. 7: Scope of anilines. The reaction is compatible with a large scope of alkyne R1substituents (aryl or alkyl). A methyl group on the alkyne is even possible (3ja). Variation of the sulfonyl group is possible. Easily removed nosyl (Ns) and 2-(trimethylsilyl)ethanesulfonyl (SES) groups are compatible with the reaction. Gratifyingly, though 2-iodo-ynamide 7 reacted a little bit less efficiently than iodoalkynes 2 with anilines 1 , a series of functionalized scaffolds 8 (for instance 8b [33] ) was obtained. Of note, a naphthyl aniline precursor could also be engaged to give adduct 8g in 48%. Fig. 8: 2-Iodo-ynamides as electrophiles. The extension of scope of alkynes 2 to the barely used 2-iodo-ynamide 7 partner proves to be possible. The corresponding products 8 offer post-functionalization opportunities. Full size image Taking advantage of the electron-richness of the ynamide moiety, we devised several transformations on polyfunctionalized substrates 8 (Fig. 9 ). While iodine smoothly promoted the formation of iodo-oxazolone 9 , a so far unknown type of derivatives, the corresponding Ag(I)-catalyzed cyclization in (wet) DCE provided the corresponding oxazolone 10 via protodesilveration [58] , [59] . Engaging the pendant aromatic ring in hydroarylation reaction was possible whether by gold(I) catalysis from 8c or by cationic rhodium catalysis [60] from the less activated substrate 8a to provide the corresponding carbazoles 10 and 12 [61] . Benzo[a]carbazoles derivatives are important structural units found in many natural products and biologically active molecules [62] , [63] as well as organic materials [64] . Fig. 9: Post-functionalizations. Ynamide-indoles 8 lend themselves to various transformation providing valuable products such as iodo-oxazolone 9 and benzo[a]carbazoles 11 and 12 . Full size image In conclusion, this study uncovers an access to 2,3-disubstituted indoles from o -alkynyl aniline derivatives via a gold-catalyzed sequence under visible-light irradiation. Subsequent to the formation of a vinylgold(I) intermediate, a photosensitized oxidative addition at gold(I) of an alkynyl iodide yields to C sp 2 -C sp cross-coupling reactions. Of note, no exogenous photocatalyst is required in these processes. On the contrary, it was found that one of the in situ formed reactant, the potassium sulfonyl amide generates emissive aggregates in the reaction medium. Variation of the temperature in the fluorescence quenching studies established a static quenching of these aggregates by the vinylgold(I) intermediate to promote its excited state. After ISC to the triplet state of the latter, reaction with an electrophile via oxidative addition and reductive elimination forges the key C-C bond. Of note, 2-iodo-ynamides could be used as electrophiles in this cross-coupling reaction. The resulting N -alkynyl indoles lend themselves to various post-functionalizations providing valuable scaffolds including benzo[a]carbazoles. The present reactant-induced photoactivation of an organogold intermediate confirms the versatility of the photosensitized oxidation process and it opens rich perspectives in the field of cross-coupling reactions for the assembly of complex frameworks. General procedure for the preparation of indoles 3 The gold(I) complex ( p -CF 3 Ph) 3 PAuCl (5 mol%), K 2 CO 3 (2.5 equiv. ), the appropriate iodoalkynes 2 (0.33 mmol, 1.1 equiv.) and o -alkynyl anilines derivatives 1 (0.3 mmol, 1.0 equiv.) 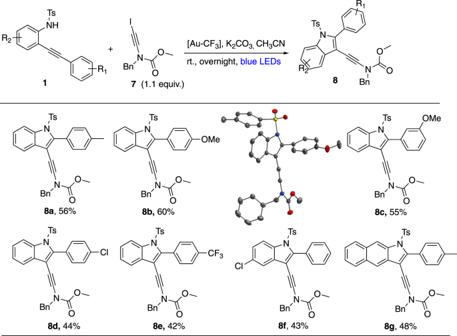Fig. 8: 2-Iodo-ynamides as electrophiles. The extension of scope of alkynes2to the barely used 2-iodo-ynamide7partner proves to be possible. The corresponding products8offer post-functionalization opportunities. 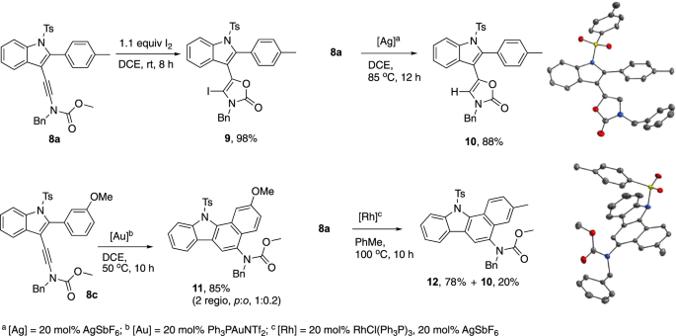Fig. 9: Post-functionalizations. Ynamide-indoles8lend themselves to various transformation providing valuable products such as iodo-oxazolone9and benzo[a]carbazoles11and12. were introduced in a Schlenk tube equipped with a magnetic stirring bar in which MeCN (4.5 ml) was added. The mixture was degassed using three freeze pump-thaw cycles and purged with argon, then irradiated with blue LEDs light for 15 h (unless mentioned). The stirring speed was equal to or more than 1200 rpm. The reaction was quenched with EtOAc (5 ml) and a 2 M HCl solution (6 ml) and the solution was extracted by EtOAc (3 × 5 ml). The combined organic layer was dried over MgSO 4 , filtered and concentrated under reduced pressure to give the crude product. The residue was purified by flash chromatography on silica gel to afford the desired product 3 .